Mitochondrial AtPAM16 is required for plant survival and the negative regulation of plant immunity Proteins containing nucleotide-binding and leucine-rich repeat domains (NB-LRRs) serve as immune receptors in plants and animals. Negative regulation of immunity mediated by NB-LRR proteins is crucial, as their overactivation often leads to autoimmunity. Here we describe a new mu tant , s nc1 - e nhancing ( muse ) forward genetic screen, targeting unknown negative regulators of NB-LRR-mediated resistance in Arabidopsis . From the screen, we identify MUSE5 , which is renamed as AtPAM16 because it encodes the ortholog of yeast PAM16, part of the mitochondrial inner membrane protein import motor. Consistently, AtPAM16–GFP localizes to the mitochondrial inner membrane. AtPAM16L is a paralog of AtPAM16 . Double mutant Atpam16-1 Atpam16l is lethal, indicating that AtPAM16 function is essential. Single mutant Atpam16 plants exhibit a smaller size and enhanced resistance against virulent pathogens. They also display elevated reactive oxygen species (ROS) accumulation. Therefore, AtPAM16 seems to be involved in importing a negative regulator of plant immunity into mitochondria, thus protecting plants from over-accumulation of ROS and preventing autoimmunity. Higher plants depend on their sophisticated immune systems to survive in nature. Two major types of immune receptors are responsible for microbial pathogen recognition and activation of downstream defence responses [1] , [2] . PAMPs (pathogen-associated molecular patterns; also known as microbe-associated molecular patterns) are recognized by plasma membrane-residing pattern recognition receptors (PRRs) to activate PAMP-triggered immunity (PTI). Successful pathogens are able to deliver specialized effectors (also termed Avirulence (Avr) proteins) into the host cell, which often perturb PTI to promote pathogen infection. On the other hand, plants have evolved resistance ( R ) genes to thwart pathogen infestation. These intracellular immune receptors recognize effectors to trigger a robust response termed effector-triggered immunity (ETI) [1] , [2] , which often includes the accumulation of the plant hormone salicylic acid (SA), induction of PATHOGENESIS-RELATED ( PR ) genes, production of reactive oxygen species (ROS) and a localized cell death referred to as the hypersensitive response (HR). As ETI is often a much stronger response compared with PTI, R protein-mediated plant immunity has a central role in defeating adapted pathogen invasion. The majority of R proteins belong to the nucleotide-binding and leucine-rich repeat (NB-LRR) class [1] , which can be further divided into two subclasses based on the presence of a Toll/Interleukin-1-receptor-like (TIR) or a coiled-coil (CC) domain at the N terminus [3] . Although many NB-LRR-encoding genes have been cloned in different plant species, it remains unclear how R proteins are activated. Arabidopsis SNC1 ( S UPPRESSOR OF N PR1-1, C ONSTITUTIVE 1 ) encodes a TIR-type NB-LRR protein [4] , [5] . In the gain-of-function mutant allele snc1 , a point mutation in the linker region between the NB and LRR results in a Glu-to-Lys change, which leads to the constitutive activation of defence responses without pathogen interaction. This mutant provides us with an ideal tool to study R protein-mediated immunity. To identify positive regulators of ETI, forward genetic suppressor screens were carried out to identify mutants that can suppress the autoimmune phenotypes of snc1 . From these screens, we identified >10 mos ( m odifier o f s nc1 ) mutations, which revealed that RNA processing, protein modification, epigenetic control of gene expression and nucleocytoplasmic trafficking are important molecular events in R protein-mediated immunity [6] . Both MOS4 and MOS2 were identified as important positive regulators from the screens. MOS4 is a component of the nuclear spliceosome-associated MOS4-associated complex, which functions in regulating the proper splicing of R genes [7] , [8] . MOS2 contains one G-patch domain and two KOW motifs and is predicted to be involved in RNA processing pathways to regulate plant immunity [9] . The success of the MOS screen exemplifies the power of the unique snc1 autoimmune model system to help dissect molecular events in ETI. In the sophisticated signalling network of plant innate immunity, negative regulators are equally important for the regulation of defence responses as overactivation of plant defence would be detrimental for plant growth and development. Here we report our newly designed snc1 enhancer screens aiming to identify negative regulators of R protein-mediated immunity. From this Mu tant, s nc1 - e nhancing (MUSE) genetic screen, we identified MUSE5 , which encodes the ortholog of the Saccharomyces cerevisiae p re-sequence translocase- a ssociated protein import m otor (PAM) subunit PAM16 of the inner mitochondrial membrane. Although mitochondria have traditionally been believed to contribute positively to plant immunity through ROS generation, our study revealed an unexpected negative regulation on mitochondria’s positive roles in plant defence. This regulation is probably achieved by a nuclear-encoded negative regulator of ROS generation, whose import into the mitochondrial matrix relies on AtPAM16. A modified snc1 enhancer screen Our previous MOS genetic screen identified positive regulators of snc1 -mediated immunity. To explore negative regulators of R protein-mediated resistance, we performed two genetic screens to search for snc1 enhancers in mos4 snc1 and mos2 snc1 npr1 backgrounds. Seeds of these two mutants, both containing a pPR2::GUS reporter gene, were mutagenized with ethyl methanesulfonate (EMS), and the M2 populations were screened for mutants that reverted to snc1 -like morphology (dwarfed size and curly leaves). A secondary screen was then carried out to select only mutants with enhanced immunity. Expression of the defence marker gene PR-2 was examined via GUS staining, and pathogen resistance was assessed by inoculating plants with the virulent oomycete Hyaloperonospora arabidopsidis ( H.a. ) Noco2. 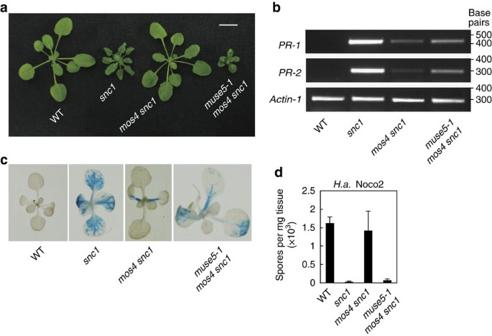Figure 1: Characterization of themuse5-1 mos4 snc1triple mutant. (a) Morphology of 3-week-old soil-grown plants of wild-type (WT),snc1,mos4 snc1andmuse5-1 mos4 snc1. Scale bar represents 1cm. (b)PR-1andPR-2expression in WT,snc1,mos4 snc1andmuse5-1 mos4 snc1as determined by RT–PCR. Total RNA was extracted from 2-week-old plants grown on 1/2 MS medium and reverse transcribed to cDNA.PR-1,PR-2andActin-1were amplified by 28 cycles of PCR using equal amounts of total cDNA, and the products were analysed by agarose gel electrophoresis followed by ethidium bromide staining. (c) GUS staining of 2-week-old plate-grown seedlings of WT,snc1,mos4 snc1andmuse5-1 mos4 snc1. All plants carry thepPR2::GUSreporter gene. (d) Quantification ofH.a.Noco2 sporulation on the indicated genotypes. Two-week-old plants were inoculated withH.a.Noco2 at a concentration of 105spores per ml of water. The spores were quantified with a hemocytometer 7 days after infection. Bars represent means±s.d. (n=4 with five plants each). Similar results were obtained in three independent experiments. Over 20 heritable mutants were obtained from the screen, which were named muse ( mu tant , s nc1 - e nhancing ) mutants ( Table 1 ). From the muse screens, we identified alleles of genes known to encode negative regulators of resistance, such as bon1 , cpr1 , siz1 , and a gain-of-function chs3-3d allele [10] ( Table 1 ). However, most of the muse mutants seem to carry mutations in novel genes that have not been studied in the past. Table 1 snc1-enhancing mutants identified from mos snc1 backgrounds. Full size table Characterization of muse5-1 mos4 snc1 The triple-mutant muse5-1 mos4 snc1 was isolated from the mutagenized mos4 snc1 population. This triple mutant reverts from the wild-type (WT)-like phenotype of mos4 snc1 to a dwarf morphology similar to snc1 ( Fig. 1a ). When the triple mutant was backcrossed with mos4 snc1 , the F1 plants were all WT-like, indicating that muse5-1 is recessive. To determine the defence phenotype of muse5-1 in the mos4 snc1 background, the expression of PR-1 and PR-2 was examined by RT–PCR. As shown in Fig. 1b , the expression of PR-1 and PR-2 was increased by muse5-1 in mos4 snc1 but not as strongly as in snc1 . Consistently, the muse5-1 mos4 snc1 plants showed much stronger pPR2::GUS staining than mos4 snc1 ( Fig. 1c ). To test whether muse5-1 alters resistance against a virulent pathogen, muse5-1 mos4 snc1 seedlings were challenged with the oomycete H.a. Noco2. As shown in Fig. 1d , the enhanced resistance response of snc1 was restored in the triple mutant. Taken together, these results show that muse5-1 enhances all aspects of snc1 -mediated autoimmunity in the mos4 snc1 background. Figure 1: Characterization of the muse5-1 mos4 snc1 triple mutant. ( a ) Morphology of 3-week-old soil-grown plants of wild-type (WT), snc1 , mos4 snc1 and muse5-1 mos4 snc1 . Scale bar represents 1cm. ( b ) PR-1 and PR-2 expression in WT, snc1 , mos4 snc1 and muse5-1 mos4 snc1 as determined by RT–PCR. Total RNA was extracted from 2-week-old plants grown on 1/2 MS medium and reverse transcribed to cDNA. PR-1 , PR-2 and Actin-1 were amplified by 28 cycles of PCR using equal amounts of total cDNA, and the products were analysed by agarose gel electrophoresis followed by ethidium bromide staining. ( c ) GUS staining of 2-week-old plate-grown seedlings of WT, snc1 , mos4 snc1 and muse5-1 mos4 snc1 . All plants carry the pPR2::GUS reporter gene. ( d ) Quantification of H.a. Noco2 sporulation on the indicated genotypes. Two-week-old plants were inoculated with H.a. Noco2 at a concentration of 10 5 spores per ml of water. The spores were quantified with a hemocytometer 7 days after infection. Bars represent means±s.d. ( n =4 with five plants each). Similar results were obtained in three independent experiments. Full size image Positional cloning of muse5-1 To identify muse5-1 , a positional cloning approach was utilized. As muse5-1 mos4 snc1 is in Columbia (Col) background, the mapping cross was carried out with the original triple mutant and Landsberg erecta ( Ler ). The F1 plants were allowed to self-fertilize and 24 F2 plants with similar morphology as muse5-1 mos4 snc1 were selected as a crude mapping population. The muse5-1 mutation was mapped to the bottom of chromosome 3 by linkage analysis and was further flanked between markers F24B22 and F2A19 using an additional 72 triple mutant-like F2 plants ( Fig. 2a ). To create a larger fine mapping population, progeny from several F2 lines heterozygous for the muse5-1 mutation and homozygous at the SNC1 locus ( snc1 ) and MOS4 locus (either WT MOS4 or mos4 ) were used to avoid interference from these two loci. Out of 383 plants from the F3 fine mapping population, 35 recombinants were collected and further analysed using markers between F24B22 and F2A19. The muse5-1 mutation was eventually mapped between markers F17J16 and T16L24, a distance of 170 kb, which was located on BAC clone F25L23 ( Fig. 2a ). To find the muse5-1 mutation, genomic DNA of plants with the muse5-1 mos4 snc1 genotypes from the mapping population was extracted and sequenced with Illumina whole-genome sequencing. After sequence comparison between the muse5-1 mutant DNA and the Arabidopsis reference genome, only one candidate mutation was found in the mapped region ( Supplementary Table S1 ). Direct Sanger sequencing of the candidate gene using muse5-1 mos4 snc1 mutant genomic DNA confirmed the G-to-A transition in At3g59280 , which occurred at an intron–exon splice junction site ( Fig. 2b ). To test whether this mutation affects the splicing pattern of At3g59280 , the cDNA of At3g59280 was amplified by RT–PCR using RNA extracted from both muse5-1 mos4 snc1 and WT plants. Comparison of the cDNA sequences of muse5-1 and the WT confirmed an aberrant splicing pattern of At3g59280 in muse5-1, resulting in a G-nucleotide deletion after the start codon ( Fig. 2c ). As a consequence of the reading frame shift, the MUSE5 protein product is no longer produced. 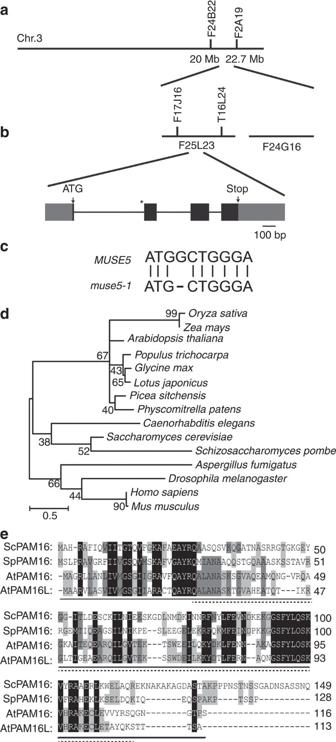Figure 2: Positional cloning ofmuse5-1. (a) Map position ofmuse5-1on chromosome 3. BAC clones are indicated. (b) Gene structure ofMUSE5(At3g59280). Boxes indicate exons and lines indicate introns. Grey regions show the UTRs. The two arrows indicate the start and stop codon, respectively. The asterisk indicates where the G-to-A mutation inmuse5-1occurred. (c) cDNA sequence comparison betweenMUSE5andmuse5-1. Inmuse5-1, one nucleotide of the third exon was spliced out due to the G-to-A mutation at the intron–exon splice junction that creates a new 3′ splice site, causing a reading frame shift. (d) Phylogenetic relationship between PAM16 and its orthologs. The orthologs are represented by the species names. Phylogenetic analysis was carried out using software MEGA v5.05. All amino acid sequences were compiled in FASTA format and used to generate alignment first. Maximum likelihood (ML) tree was implemented assessing with 1,000 bootstrap replications. (e) Full-length amino acid sequence alignments of MUSE5, MUSE5L and PAM16 proteins fromS. cerevisiae(Sc) andS. pombe(Sp). The conserved PAM16 domain and degenerate J domain (J-like domain) are underlined by solid and dotted lines, respectively. Black boxes indicate regions in which at least two of three residues are identical and grey boxes indicate conserved residues. Figure 2: Positional cloning of muse5-1 . ( a ) Map position of muse5-1 on chromosome 3. BAC clones are indicated. ( b ) Gene structure of MUSE5 ( At3g59280 ). Boxes indicate exons and lines indicate introns. Grey regions show the UTRs. The two arrows indicate the start and stop codon, respectively. The asterisk indicates where the G-to-A mutation in muse5-1 occurred. ( c ) cDNA sequence comparison between MUSE5 and muse5-1 . In muse5-1 , one nucleotide of the third exon was spliced out due to the G-to-A mutation at the intron–exon splice junction that creates a new 3′ splice site, causing a reading frame shift. ( d ) Phylogenetic relationship between PAM16 and its orthologs. The orthologs are represented by the species names. Phylogenetic analysis was carried out using software MEGA v5.05. All amino acid sequences were compiled in FASTA format and used to generate alignment first. Maximum likelihood (ML) tree was implemented assessing with 1,000 bootstrap replications. ( e ) Full-length amino acid sequence alignments of MUSE5, MUSE5L and PAM16 proteins from S. cerevisiae (Sc) and S. pombe (Sp). The conserved PAM16 domain and degenerate J domain (J-like domain) are underlined by solid and dotted lines, respectively. Black boxes indicate regions in which at least two of three residues are identical and grey boxes indicate conserved residues. Full size image MUSE5 is a small conserved protein that belongs to the DnaJ chaperon superfamily ( Fig. 2d ). There is one predicted paralog of MUSE5 ( At5g61880 , named MUSE5L ) in Arabidopsis . MUSE5 shares 35% amino-acid sequence identity to the S. cerevisiae P re-sequence translocase- a ssociated protein import m otor (PAM) subunit PAM16. Alignment of MUSE5, MUSE5L and PAM16 displays the highly conserved PAM16 domain of the proteins ( Fig. 2e ). Within the PAM16 domain, there is a region of ~85 residues that is denoted as J-like domain ( Fig. 2e ), which has been shown to be responsible for dimerization with the J domain of PAM18 (refs 11 , 12 ). Confirmation that MUSE5 is At3g59280 Transgenic complementation was carried out to confirm whether the mutation found in At3g59280 ( Fig. 2b ) is responsible for enhancing the snc1 mutant phenotypes. Full-length At3g59280 genomic DNA containing 1,067 bp sequence before the start codon was PCR-amplified from WT plants and cloned into a binary vector, which was then transformed into the muse5-1 mos4 snc1 triple mutant. Six independent transgenic lines all displayed mos4 snc1 -like morphology. Two representative plants from line #1 and #2 are shown in Fig. 3a . These transgenic plants are slightly smaller than mos4 snc1 as quantified by whole-plant fresh weight analysis ( Fig. 3b ). When inoculated with H.a. Noco2, these transgenic plants displayed elevated susceptibility as compared with muse5-1 mos4 snc1 ( Fig. 3c ). The intermediate phenotypes of these transgenic plants demonstrate that wild-type At3g59280 can mostly but not fully complement the muse5-1 defects. This could be due to the missing unknown regulatory elements that were not included in the genomic construct of At3g59280 . 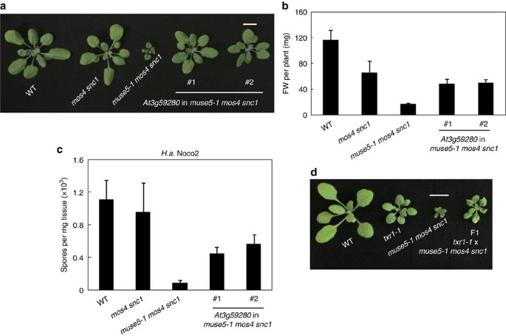Figure 3: Confirmation thatMUSE5isAt3g59280. (a) Plant morphology of WT,mos4 snc1,muse5-1 mos4 snc1andmuse5-1 mos4 snc1transformed with a genomic clone ofAt3g59280. Two representative homozygous T3 plants from independent transgenic events are shown. Scale bar is 1 cm. (b) Fresh weight (FW) of plants of the indicated genotypes when they are 3-week-old. Bars represent means±s.d. (n=12). The experiments were repeated three times with similar results. (c) Quantification ofH.a.Noco2 sporulation on the same genotypes as (a). Ten-day-old plants were sprayed withH.a.Noco2 at a concentration of 105spores per ml of water. The oomycete spores on the surface of leaves were quantified seven days after inoculation. Bars represent means±s.d. (n=4 with five plants each). Three independent experiments were carried out and similar results were obtained. (d) Morphology of plants from the allelism test betweentxr1-1andmuse5-1. F1 was generated from the cross betweentxr1-1single mutant andmuse5-1 mos4 snc1triple mutant. Scale bar is 1 cm. Figure 3: Confirmation that MUSE5 is At3g59280 . ( a ) Plant morphology of WT, mos4 snc1 , muse5-1 mos4 snc1 and muse5-1 mos4 snc1 transformed with a genomic clone of At3g59280 . Two representative homozygous T3 plants from independent transgenic events are shown. Scale bar is 1 cm. ( b ) Fresh weight (FW) of plants of the indicated genotypes when they are 3-week-old. Bars represent means±s.d. ( n =12). The experiments were repeated three times with similar results. ( c ) Quantification of H.a. Noco2 sporulation on the same genotypes as ( a ). Ten-day-old plants were sprayed with H.a. Noco2 at a concentration of 10 5 spores per ml of water. The oomycete spores on the surface of leaves were quantified seven days after inoculation. Bars represent means±s.d. ( n =4 with five plants each). Three independent experiments were carried out and similar results were obtained. ( d ) Morphology of plants from the allelism test between txr1-1 and muse5-1 . F1 was generated from the cross between txr1-1 single mutant and muse5-1 mos4 snc1 triple mutant. Scale bar is 1 cm. Full size image Previously, At3g59280 was named T ha X tomin R esistant 1 ( TXR1 ) as mutants of this gene exhibit insensitivity to the cellulose synthesis inhibitor thaxtomin [13] . When we crossed txr1-1 with muse5-1 mos4 snc1 , heterozygous F1 plants exhibited snc1 -like phenotype ( Fig. 3d ), indicating that muse5-1 failed to complement txr1-1 . Taken together, our data suggest that MUSE5 is At3g59280 / TXR1 . At3g59280/TXR1/MUSE5 is an ortholog of yeast PAM16 TXR1/MUSE5 shares 35% amino-acid sequence identity to the S. cerevisiae PAM16 ( Fig. 2e ), which is a small protein of the inner mitochondrial membrane that is conserved in all fully sequenced eukaryotic genomes. There are two predicted PAM16 paralogs in Arabidopsis , At3g59280/MUSE5/TXR1 and At5g61880 . Previously, PAM16, the fifth identified subunit of the PAM, was found to be essential in driving preprotein import into the mitochondrial matrix in S. cerevisiae [12] . Thus, a yeast complementation experiment was carried out to determine whether MUSE5 is orthologous to PAM16. The pam16-1 allele is a temperature-conditional partial loss-of-function yeast strain generated by error-prone PCR, which grows like the wild-type strain at 30 °C but does not grow at 37 °C. At 37 °C, only WT and pam16-1 cells expressing TXR1/MUSE5 can grow ( Fig. 4a ), suggesting that TXR1 / MUSE5 can fully complement the yeast pam16-1 mutant phenotype. To test whether the yeast PAM16 is also able to complement muse5 , we cloned yeast PAM16 and stably expressed it under the control of 35S promoter in muse5-1 mos4 snc1 triple mutant. As shown in Fig. 4b , the representative transgenic plants revert from muse5-1 mos4 snc1 to mos4 snc1 -like morphology. This complementing phenotype indicates that the yeast PAM16 and MUSE5 are indeed orthologous. As TXR1/MUSE5 is an ortholog of yeast PAM16 , we renamed At3g59280 as AtPAM16 and At5g61880 as AtPAM16L . The muse5-1 allele is renamed Atpam16-1 , and txr1-1 is renamed Atpam16-2 . 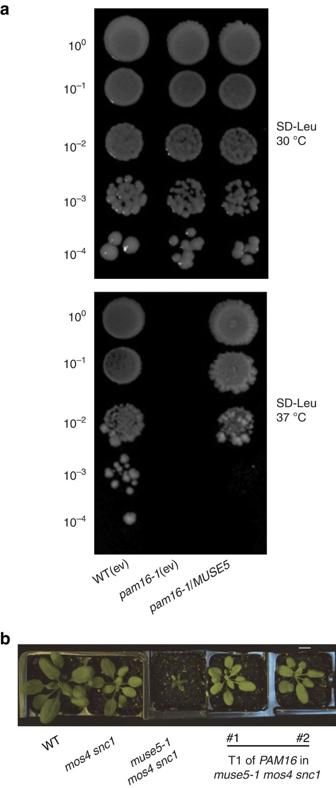Figure 4:AtPAM16and yeastPAM16can complement each other across kingdoms. (a) Serial 1/10 dilutions of the following yeast strains containing the same number of cells were plated on SD-Leu medium: left lane, the wild-type (WT) strain expressing empty vector (ev); middle lane,pam16-1partial loss-of-function strain expressing empty vector; right lane,pam16-1knockout strain expressingAtPAM16. Yeast plates were incubated for 3 days at the indicated temperatures before the picture was taken. (b) Morphology of WT,mos4 snc1,muse5-1 mos4 snc1and two representative transgenic T1 plants ofmuse5-1 mos4 snc1transformed with35S-PAM16. The plants were 4 weeks old when the picture was taken. Scale bar represents 1 cm. Figure 4: AtPAM16 and yeast PAM16 can complement each other across kingdoms. ( a ) Serial 1/10 dilutions of the following yeast strains containing the same number of cells were plated on SD-Leu medium: left lane, the wild-type (WT) strain expressing empty vector (ev); middle lane, pam16-1 partial loss-of-function strain expressing empty vector; right lane, pam16-1 knockout strain expressing AtPAM16 . Yeast plates were incubated for 3 days at the indicated temperatures before the picture was taken. ( b ) Morphology of WT, mos4 snc1 , muse5-1 mos4 snc1 and two representative transgenic T1 plants of muse5-1 mos4 snc1 transformed with 35S-PAM16 . The plants were 4 weeks old when the picture was taken. Scale bar represents 1 cm. Full size image AtPAM16 localizes to mitochondrial inner membrane To identify the subcellular localization of AtPAM16, a construct containing full-length genomic AtPAM16 DNA, fused with GFP at its C terminus and driven by its endogenous promoter containing 1,067 bp sequence before the start codon, was transformed into the Atpam16-1 mos4 snc1 triple mutant. Similar to expressing AtPAM16 :: AtPAM16 in the triple background ( Fig. 3 ), expressing AtPAM16 :: AtPAM16–GFP in all 12 transgenic lines also mostly complemented the defects of the triple mutant, suggesting that AtPAM16–GFP is functional, although the plants are slightly smaller than mos4 snc1 ( Fig. 5a,b ). These transgenic plants displayed similar susceptibility to H.a. Noco2 as compared with mos4 snc1 ( Fig. 5c ). To investigate the subcellular localization of AtPAM16–GFP in vivo , we analysed leaf and root tissues of the transgenic plants by confocal laser scanning microscopy (CLSM). Green fluorescent protein (GFP) fluorescence in both leaf and root cells was observed in punctate structures ( Fig. 5d ). According to the size and dynamic movement of the AtPAM16–GFP signals within the cells, they are likely to be mitochondria. To confirm mitochondrial localization of AtPAM16, we crossed the transgenic AtPAM16–GFP lines with an established mitochondrial marker line stably expressing CFP fused to a mitochondrial targeting sequence (the first 29 amino acids of S. cerevisiae cytochrome c oxidase IV; mt-ck CS16262 ) [14] . AtPAM16–GFP fluorescence was found to colocalize with mitochondria-targeted CFP (mt-CFP in Fig. 5e ) when root cells of F1 plants were examined by CLSM ( Fig. 5e ). Interestingly, at this higher magnification increased fluorescence was observed at the rim of mitochondria, indicating membrane localization ( Fig. 5e ). 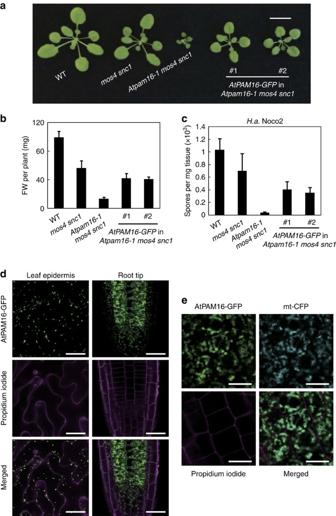Figure 5: AtPAM16–GFP localizes to the mitochondrial membrane. (a) Morphology of WT,mos4 snc1,Atpam16-1 mos4 snc1andAtpam16-1 mos4 snc1transformed withAtPAM16–GFP. Two representative homozygous T3 plants from independent transgenic lines are shown. Scale bar is 1 cm. (b) Fresh weight (FW) of 3-week-old plants of the indicated genotypes. Bars represent means±s.d. (n=12). The experiments were repeated three times with similar results. (c) Quantification ofH.a.Noco2 sporulation on the same genotypes asFig. 5a. Ten-day-old seedlings were inoculated with a conidiospore suspension of 105spores per ml of water. Spores were counted 1 week after inoculation. Bars represent means±s.d. (n=4 with 5 plants each). Three independent experiments were carried out with similar results. (d) Confocal images of AtPAM16–GFP fluorescence in leaf pavement and root cells of soil-grownAtpam16-1 mos4 snc1transgenic plants expressingAtPAM16–GFPunder control of the nativeAtPAM16promoter. Cell walls were stained with propidium iodide to visualize the outlines of cells. Scale bars are 20 μm. (e) AtPAM16–GFP colocalizes with CFP fused to a mitochondrial targeting sequence. Confocal fluorescence microscopy images of root cells of soil-grown F1plants grown from a cross between a transgenic plant expressingAtPAM16–GFPunder its native promoter in theAtpam16-1 mos4 snc1background and a transgenic marker line expressing CFP fused to a 29-amino acid mitochondrial (mt) targeting sequence ofS. cerevisiaecytochromecoxidase IV14. Cell walls were stained with propidium iodide to visualize the outlines of cells. Scale bars are 10 μm. At this higher magnification, the image is a bit blurry due to fast movements of the mitochondria. Figure 5: AtPAM16–GFP localizes to the mitochondrial membrane. ( a ) Morphology of WT, mos4 snc1 , Atpam16-1 mos4 snc1 and Atpam16-1 mos4 snc1 transformed with AtPAM16 – GFP . Two representative homozygous T3 plants from independent transgenic lines are shown. Scale bar is 1 cm. ( b ) Fresh weight (FW) of 3-week-old plants of the indicated genotypes. Bars represent means±s.d. ( n =12). The experiments were repeated three times with similar results. ( c ) Quantification of H.a. Noco2 sporulation on the same genotypes as Fig. 5a . Ten-day-old seedlings were inoculated with a conidiospore suspension of 10 5 spores per ml of water. Spores were counted 1 week after inoculation. Bars represent means±s.d. ( n =4 with 5 plants each). Three independent experiments were carried out with similar results. ( d ) Confocal images of AtPAM16–GFP fluorescence in leaf pavement and root cells of soil-grown Atpam16-1 mos4 snc1 transgenic plants expressing AtPAM16–GFP under control of the native AtPAM16 promoter. Cell walls were stained with propidium iodide to visualize the outlines of cells. Scale bars are 20 μm. ( e ) AtPAM16–GFP colocalizes with CFP fused to a mitochondrial targeting sequence. Confocal fluorescence microscopy images of root cells of soil-grown F 1 plants grown from a cross between a transgenic plant expressing AtPAM16–GFP under its native promoter in the Atpam16-1 mos4 snc1 background and a transgenic marker line expressing CFP fused to a 29-amino acid mitochondrial (mt) targeting sequence of S. cerevisiae cytochrome c oxidase IV [14] . Cell walls were stained with propidium iodide to visualize the outlines of cells. Scale bars are 10 μm. At this higher magnification, the image is a bit blurry due to fast movements of the mitochondria. Full size image To test whether AtPAM16–GFP localizes to the inner mitochondrial membrane as does yeast PAM16, we utilized two independent strategies, a biochemical proteinase K digestion assay and a transmission electron microscopy (TEM) immuno-gold labeling approach using seedlings expressing the native promoter-driven AtPAM16 – GFP . As shown in Fig. 6a , when isolated intact mitochondria were treated with proteinase K, AtPAM16–GFP was resistant to digestion. However, when the same mitochondria were disrupted by sonication, AtPAM16–GFP could be readily degraded upon proteinase K treatment, as could the mitochondrial inner membrane protein cytochrome c . This suggests that AtPAM16–GFP is protected from proteinase K digestion because it is localized inside the mitochondria. In addition, when the same transgenic plants were cryofixed, freeze-substituted and immunolabeled for TEM, quantification of AtPAM16–GPF signal, as detected by a gold-conjugated anti-GFP antibody, revealed significantly more label on mitochondria (mean±s.e.=0.00969±0.00064, gold μm −2 ) as compared with other cellular components (cytoplasm, other organelles, cell wall=0.00253±0.00016, gold μm −2 ) in AtPAM16–GPF expressing seedlings, or compared with background signal detected in WT samples not expressing the AtPAM16 – GFP transgene (ANOVA, P <0.0001, n =81 measurements for AtPAM16–GFP, 94 measurements for WT; Fig. 6b,c ). This mitochondrial signal was not detected in WT seedlings without the AtPAM16 – GFP transgene ( Fig. 6d ) or in AtPAM16 – GFP seedlings treated without the primary antibody as a control ( Fig. 6e ). 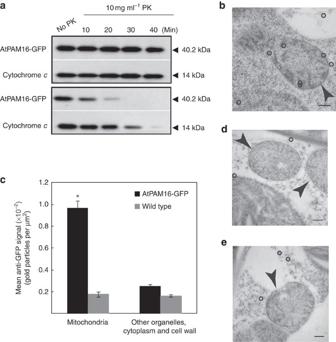Figure 6: AtPAM16–GFP localizes to mitochondria inner membrane. (a) Immunodetection of AtPAM16–GFP from isolated mitochondria treated with proteinase K. Intact mitochondria (top panel) or sonication-ruptured mitochondria (lower panel) were treated with 10 mg ml−1proteinase K (PK). Cytochromec, a known mitochondria inner membrane protein, was used as positive control. (b) Immuno-TEM using a gold-conjugated anti-GFP antibody to detect AtPAM16–GFP. Arrowhead points to mitochondrion, circles highlight gold particles, scale bar represents 200 nm. (c) Quantification of mitochondrial signal relative to background signal in cytoplasm, other organelles and the cell wall revealed significantly more gold per μm2in mitochondria (ANOVA,P<0.0001,n=81 AtPAM16–GFP,n=94 wild type). * indicates a statistically significant difference, error bars represent s.e. (d) Col-0 seedlings without the AtPAM16–GFP transgene treated with anti-GFP. Arrowheads point to mitochondria, circles highlight gold particles, and scale bar represents 200 nm. (e) The AtPAM16–GFP inner mitochondrial membrane signal was not detected in AtPAM16–GFP seedlings treated without a primary antibody. Arrowhead points to mitochondrion, circles highlight gold particles and scale bar represents 200 nm. Figure 6: AtPAM16–GFP localizes to mitochondria inner membrane. ( a ) Immunodetection of AtPAM16–GFP from isolated mitochondria treated with proteinase K. Intact mitochondria (top panel) or sonication-ruptured mitochondria (lower panel) were treated with 10 mg ml −1 proteinase K (PK). Cytochrome c , a known mitochondria inner membrane protein, was used as positive control. ( b ) Immuno-TEM using a gold-conjugated anti-GFP antibody to detect AtPAM16–GFP. Arrowhead points to mitochondrion, circles highlight gold particles, scale bar represents 200 nm. ( c ) Quantification of mitochondrial signal relative to background signal in cytoplasm, other organelles and the cell wall revealed significantly more gold per μm 2 in mitochondria (ANOVA, P <0.0001, n =81 AtPAM16–GFP, n =94 wild type). * indicates a statistically significant difference, error bars represent s.e. ( d ) Col-0 seedlings without the AtPAM16–GFP transgene treated with anti-GFP. Arrowheads point to mitochondria, circles highlight gold particles, and scale bar represents 200 nm. ( e ) The AtPAM16–GFP inner mitochondrial membrane signal was not detected in AtPAM16–GFP seedlings treated without a primary antibody. Arrowhead points to mitochondrion, circles highlight gold particles and scale bar represents 200 nm. Full size image Taken together, our data suggest that AtPAM16 localizes to the inner membrane of mitochondria like its yeast ortholog PAM16. Analysis of Atpam16 single mutants From the snc1 -enhancing phenotypes of Atpam16-1 , we deduced that AtPAM16 probably serves as a negative regulator of snc1 -mediated immunity. To determine its function in the absence of the snc1 mutation, we analysed the phenotypes of Atpam16-1 ( muse5-1 ), Atpam16-2 ( txr1-1 ) and Atpam16l ( At5g61880 ) single mutants. The Atpam16-1 single mutant was obtained from the F2 generation of a cross between Atpam16-1 mos4 snc1 and WT. We also obtained a T-DNA insertion mutant allele of AtPAM16L , which is homologous to AtPAM16 with 73% similarity ( Fig. 2e ). This T-DNA mutant (SALK_061634C) contains an insertion in the second exon of AtPAM16L , likely leading to truncation of the encoded protein. Compared with WT, Atpam16-1 and Atpam16-2 displayed smaller size whereas Atpam16l exhibit no obvious morphological defects ( Fig. 7a ). Atpam16-2 plants are consistently slightly smaller than Atpam16-1 plants, suggesting that Atpam16-2 is a stronger allele than Atpam16-1 . Single mutant Atpam16-1 , Atpam16-2 and Atpam16l plants were slightly more resistant to H.a. Noco2 compared with WT ( Fig. 7b ). In addition, when challenged with virulent bacterial pathogen Pseudomonas syringae pv. maculicola ( P.s.m. ) ES4326, both Atpam16-1 and Atpam16-2 exhibit enhanced resistance compared with WT, whereas the susceptibility of Atpam16l is similar to WT ( Fig. 7c ). The relative expression levels of PR-1 and PR-2 in these three single mutants were constitutively higher than those in WT ( Fig. 7d ), with Atpam16-2 showing the highest expression of these defence marker genes. Taken together, these results indicate that mutations in AtPAM16 cause enhanced disease resistance. 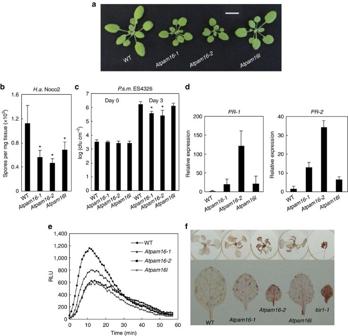Figure 7: Single mutant analysis ofAtpam16andAtpam16l. (a) Morphology of WT,Atpam16-1,Atpam16-2andAtpam16lsingle mutants. The picture was taken from soil-grown plants when they were 3 weeks old. Scale bar represents 1 cm. (b) Quantification ofH.a.Noco2 sporulation in WT,Atpam16-1,Atpam16-2andAtpam16lseedlings. Two-week-old plants were inoculated withH.a.Noco2 at a concentration of 105spores per ml of water. The oomycete spores on the surface of leaves were counted 7 days after inoculation. Bars represent means±s.d. (n=4 with 5 plants each). The experiment was repeated three times and similar results were observed. Asterisks indicate significant differences ofAtpam16-1,Atpam16-2andAtpam16lcompared with WT based on Student’sttest,P<0.05 (*). (c) Bacterial growth ofP.s.m.ES4326 in WT,Atpam16-1,Atpam16-2andAtpam16l. Leaves of 4-week-old plants were infiltrated with a bacterial suspension at OD600=0.0005. Leaf discs within the infected area were taken at day 0 and day 3 to quantify colony-forming units (CFU). Bars represent means±s.d. (n=5). Asterisks indicate significant differences ofAtpam16-1,Atpam16-2andAtpam16lcompared with WT based on Student’sttest,P<0.05 (*). (d) Relative expression ofPR-1andPR-2in WT,Atpam16-1,Atpam16-2andAtpam16las determined by real-time RT–PCR. Total RNA was extracted from 4-week-old plants grown on soil and reverse transcribed to cDNA. BothPR-1andPR-2expression levels were normalized byActin-1. Bars represent means±s.d. (n=3). The experiment was repeated three times with similar results. (e) Oxidative burst in response to flg22 in WT,Atpam16-1,Atpam16-2andAtpam16l. Under 12 h light/12 h dark cycle growth condition, leaf slices of 4-week-old plants were treated with 1 μM flg22 as elicitor. Oxidative burst was indirectly measured as relative light units (RLU) using a luminol-based chemiluminescence assay38. Three independent experiments (n=10) were performed with similar results. (f) DAB staining of 2-week-old 1/2 MS plate-grown plants of WT,Atpam16-1,Atpam16-2andAtpam16l. The whole plants and representative leaves are shown. Mutantbir1-1was used as positive control. Figure 7: Single mutant analysis of Atpam16 and Atpam16l . ( a ) Morphology of WT, Atpam16-1 , Atpam16-2 and Atpam16l single mutants. The picture was taken from soil-grown plants when they were 3 weeks old. Scale bar represents 1 cm. ( b ) Quantification of H.a. Noco2 sporulation in WT, Atpam16-1 , Atpam16-2 and Atpam16l seedlings. Two-week-old plants were inoculated with H.a. Noco2 at a concentration of 10 5 spores per ml of water. The oomycete spores on the surface of leaves were counted 7 days after inoculation. Bars represent means±s.d. ( n =4 with 5 plants each). The experiment was repeated three times and similar results were observed. Asterisks indicate significant differences of Atpam16-1 , Atpam16-2 and Atpam16l compared with WT based on Student’s t test, P <0.05 (*). ( c ) Bacterial growth of P.s.m. ES4326 in WT, Atpam16-1 , Atpam16-2 and Atpam16l . Leaves of 4-week-old plants were infiltrated with a bacterial suspension at OD 600 =0.0005. Leaf discs within the infected area were taken at day 0 and day 3 to quantify colony-forming units (CFU). Bars represent means±s.d. ( n =5). Asterisks indicate significant differences of Atpam16-1 , Atpam16-2 and Atpam16l compared with WT based on Student’s t test, P <0.05 (*). ( d ) Relative expression of PR-1 and PR-2 in WT, Atpam16-1 , Atpam16-2 and Atpam16l as determined by real-time RT–PCR. Total RNA was extracted from 4-week-old plants grown on soil and reverse transcribed to cDNA. Both PR-1 and PR-2 expression levels were normalized by Actin-1 . Bars represent means±s.d. ( n =3). The experiment was repeated three times with similar results. ( e ) Oxidative burst in response to flg22 in WT, Atpam16-1 , Atpam16-2 and Atpam16l . Under 12 h light/12 h dark cycle growth condition, leaf slices of 4-week-old plants were treated with 1 μM flg22 as elicitor. Oxidative burst was indirectly measured as relative light units (RLU) using a luminol-based chemiluminescence assay [38] . Three independent experiments ( n =10) were performed with similar results. ( f ) DAB staining of 2-week-old 1/2 MS plate-grown plants of WT, Atpam16-1 , Atpam16-2 and Atpam16l . The whole plants and representative leaves are shown. Mutant bir1-1 was used as positive control. Full size image Mitochondria are sites of ROS production, which is believed to contribute to R protein-mediated immune responses. As AtPAM16 is part of the import motor of mitochondria, we examined ROS levels in the Atpam16 mutants via luminol-based chemiluminescence assay and DAB staining. As shown in Fig. 7e , upon flg22 PAMP peptide treatment, both alleles of Atpam16 exhibited higher ROS levels compared with WT and Atpam16l , with Atpam16-2 showing the highest ROS production. A similar trend was observed with DAB staining. Mutant bir1-1 seedlings were used as positive control, as the mutant accumulates very high levels of hydrogen peroxide, resulting in strong DAB staining [15] . Obvious darker brown staining was observed on Atpam16-2 seedlings compared with WT ( Fig. 7f ). The staining is weaker in Atpam16-1 , consistent with it being a weaker mutant allele of AtPAM16 . Atpam16l displayed much fainter staining that is comparable to that of WT. We tried to create an Atpam16-1 Atpam16l double mutant. Although 200 F2 plants from the cross between Atpam16-1 and Atpam16l were genotyped to screen for the double mutant, no Atpam16-1 Atpam16l double mutant could be identified. In the F3 generation obtained from 12 F2 plants heterozygous for Atpam16-1 and homozygous for Atpam16l , we still could not obtain the double mutant, indicating that the double mutant is lethal. As PAM16 is part of the mitochondrial protein import motor, these data suggest that mitochondrial protein import is essential for regular plant development and survival. The lethality of the double mutant also indicates that AtPAM16 and AtPAM16L function redundantly, with AtPAM16 having a more dominant role in plant immunity as compared with its paralog AtPAM16L . Only Atpam16-1 and Atpam16-2 can enhance snc1 -mediated immunity To further test the enhancing impact of AtPAM16 mutations on snc1 -mediated immune responses, Atpam16-1 snc1 , Atpam16-2 snc1 and Atpam16l snc1 double mutants were generated. Both Atpam16-1 snc1 and Atpam16-2 snc1 exhibited snc1 -enhancing stunted growth compared with snc1 , whereas Atpam16l snc1 is indistinguishable from snc1 ( Fig. 8a ). All three double mutants were more resistant to the oomycete pathogen H.a. Noco2 compared with WT ( Fig. 8b ). Thus, snc1 -mediated immune response can only be enhanced by Atpam16-1 and Atpam16-2 , but not by Atpam16l. 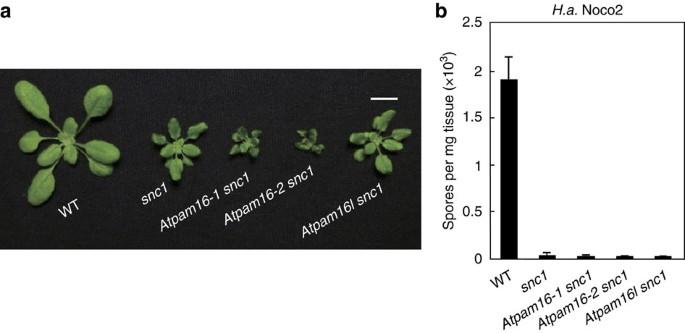Figure 8: Analysis ofAtpam16 snc1double mutants. (a) Plant morphology of WT,snc1,Atpam16-1 snc1,Atpam16-2 snc1andAtpam16l snc1. The picture was taken of soil-grown plants when they were 3 weeks old. Scale bar is 1 cm. (b) Quantification ofH.a.Noco2 sporulation in WT,snc1,Atpam16-1 snc1,Atpam16-2 snc1andAtpam16l snc1seedlings. Two-week-old seedlings were sprayed withH.a.Noco2 at a concentration of 105spores per ml of water. The spores were quantified 1 week after infection. Bars represent means±s.d. (n=4 with five plants each). Similar results were observed in three independent experiments. Figure 8: Analysis of Atpam16 snc1 double mutants. ( a ) Plant morphology of WT, snc1 , Atpam16-1 snc1 , Atpam16-2 snc1 and Atpam16l snc1 . The picture was taken of soil-grown plants when they were 3 weeks old. Scale bar is 1 cm. ( b ) Quantification of H.a. Noco2 sporulation in WT, snc1 , Atpam16-1 snc1 , Atpam16-2 snc1 and Atpam16l snc1 seedlings. Two-week-old seedlings were sprayed with H.a. Noco2 at a concentration of 10 5 spores per ml of water. The spores were quantified 1 week after infection. Bars represent means±s.d. ( n =4 with five plants each). Similar results were observed in three independent experiments. Full size image During the past two decades, many genetic screens have been targeting towards finding negative regulators of plant immunity. For example, early screens aiming at the isolation of mutants showing accelerated cell death (ACD) and lesions simulating disease (LSD) resistance identified components that are responsible for cell death or HR suppression [16] , [17] . Additional mutations in negative regulators were identified from defence marker-assisted screens such as the constitutive expression of PR genes (CPR) screen using pPR2-GUS and the constitutive immunity (CIM) screen based on the pPR1 -luciferase reporter activity [18] , [19] . Suppressor screens with different npr1 mutant alleles were independently carried out in suppressor of npr1 , inducible (SNI), suppressor of npr1 , constitutive (SNC) and suppressor of SA insensitivity (SSI) screens, which identified a number of negative regulators dependent or independent of NPR1 (refs 4 , 20 , 21 , 22 ). Although these screens have been exhaustive in generating mutants that exhibit extreme constitutive immune responses, such as lesion mimic or extremely dwarfed plants, negative regulators that do not exhibit severe morphological defects when mutated have not been targeted using a genetic approach. This is partly due to technical difficulties in identifying the mutation with traditional map-based cloning approaches. Here, we describe our mu tant, s nc1 - e nhancing (MUSE) genetic screen, intending to identify negative regulators that do not necessarily show dramatic autoimmunity defects when mutated. This screen is a modified version of a snc1 enhancer screen in which we are particularly interested in mutants that show minor phenotypes by themselves, but are able to drastically enhance snc1 -mediated autoimmunity. These mutants may reveal a large number of missing negative regulators in plant immune regulatory pathways. The usage of the unique snc1 mutant not only provides us with a sensitized background to reveal mild enhanced-resistance phenotypes of the muse mutants, it also enables convenient phenotyping during further genetic mapping. In order to avoid possible lethality of the snc1 muse double mutants due to enhanced autoimmunity, we utilized plants with mos2 or mos4 in the snc1 background that grow to wild-type size and morphology despite the snc1 mutation [7] , [9] . As a proof of concept, we identified several mutant alleles of three well-known negative regulators of plant immunity, BON1 , CPR1 and SIZ1 ( Table 1 ). We also identified a rare gain-of-function chs3-3d allele [10] and several intragenic second-site gain-of-function alleles of snc1 , which will be reported elsewhere. Both BON1 and CPR1 are genetically dependent on SNC1 [23] , [24] , [25] . BON1 regulates SNC1 transcription through unknown mechanisms, whereas SCF CPR1 directly targets SNC1 and other NB-LRR proteins for degradation [24] , [25] . The SUMO E3 ligase SIZ1 is involved in the regulation of many biological processes, one of which is the negative regulation of defence hormone salicylic acid (SA) accumulation [26] , [27] . However, the exact role of SIZ1 in the regulation of SA signalling is unclear. Aside from these known negative regulators of plant immunity, most of the muse mutants we identified so far seem to carry mutations in novel genes as they do not map to known negative regulators of plant disease resistance. Future cloning and detailed biochemical studies of these MUSE genes and their encoded proteins, one of which (MUSE5/AtPAM16) is described here, will enable us to better understand negative regulatory mechanisms that help fine-tune plant immunity. Much of the mitochondrial protein import mechanism has been uncovered from studies using yeast. In eukaryotes, >98% of mitochondrial proteins are nuclear-encoded and ~10–15% of nuclear genes encode mitochondrial proteins that need to be either incorporated into the organelle membrane or imported into the matrix. Proteins targeted to the mitochondrial matrix need to be transported by two distinct transport machineries. The TOM complex transfers proteins across the mitochondrial outer membrane, whereas the TIM23 complex transports the protein through the inner membrane [28] , [29] . PAM16 is part of the import motor of the TIM23 complex that facilitates the import of preproteins together with the mtHSP70 proteins and the co-chaperones Mge1, Tim44 and Pam18. It forms a stable heterodimer with PAM18 and resides on the matrix-side of the mitochondrial inner membrane [30] . In yeast pam16 mutants, preprotein import into the matrix is defective [12] . The analogous and vital preprotein import function of PAM16 in Arabidopsis is supported by our data that Atpam16 Atpam16l double mutant plants are lethal. The conservation of the mitochondrial protein import machinery is also reflected by the fact that most of the TOM and TIM23 complex member-encoding genes can be found in Arabidopsis and other higher eukaryotes. Using a combination of traditional mapping and next-generation sequencing, we identified MUSE5 as AtPAM16 . Several lines of evidence indicate that AtPAM16 is an ortholog of the yeast mitochondrial inner membrane protein import motor PAM16. First, AtPAM16 is able to fully complement a yeast temperature-conditional pam16 allele ( Fig. 4a ), while the yeast PAM16 is able to complement Atpam16 defects ( Fig. 4b ). These complementation data indicate that PAM16 is functionally highly conserved among eukaryotes, agreeing with the sequence analysis of PAM16 -encoding genes in different organisms ( Fig. 2d ). Additionally, in Arabidopsis , expression of the AtPAM16–GFP fusion gene construct complements the Atpam16 defects, suggesting that the fusion protein localizes to the proper subcellular compartment. Indeed, confocal fluorescence microscopy confirmed that AtPAM16–GFP localizes to mitochondrial rims ( Fig. 5d,e ), supporting its predicted function as part of the mitochondrial inner membrane protein import motor. In addition, our cryo-TEM and proteinase K digestion assay suggest that AtPAM16 indeed localizes to the inner membrane of mitochondria ( Fig. 6a–c ). Previously, an Atpam16-2 mutant allele (named txr1-1 ) was identified from a forward genetic screen searching for thaxtomin A-resistant mutants [13] . Thaxtomin A is a phytotoxin from Streptomyces species, in particular Streptomyces scabies , the causal agent of potato scab. Application of thaxtomin A at a concentration as low as 50 nM causes Arabidopsis seedlings to exhibit severe growth retardation as a consequence of cellulose synthesis inhibition [13] . The strong effect of thaxtomin A on cellulose synthesis is intriguing [13] , [31] . One interesting observation Bischoff et al. [31] made is that application of thaxtomin enhances PR gene expression (Fig. 2 in the study of Bischoff et al. [31] ), which is in agreement with the heightened PR gene expression of Atpam16 mutants ( Fig. 7d ). As our analysis revealed that TXR1 is actually AtPAM16, an alternative model of thaxtomin A’s mode of action is proposed. It is possible that the cellulose synthesis defects are downstream of its primary toxicity on mitochondria. Thaxtomin A may be targeting a mitochondrial matrix protein that relies on AtPAM16 for import or it could be directly targeting AtPAM16 itself. Such targeting may serve as a virulence strategy to release a death signal from mitochondria and assists the killing of host cells so that the pathogen can consume the plant’s photosynthates. The thaxtomin-resistant phenotype of Atpam16 mutant plants is in agreement with this hypothesis. In Atpam16 mutant plants, this thaxtomin target may no longer be effectively imported into the matrix, thus exhibiting a thaxtomin-resistant phenotype. Future analysis on the effect of the phytotoxin on mitochondria will reveal more accurate relationships between the two. How does AtPAM16 as part of the mitochondrial inner membrane import motor regulate plant immunity? Mitochondria have long been connected with the HR, a programmed cell death event that is associated with R protein-mediated immunity. It has been shown that mitochondria release the death signal cytochrome c to the cytosol, leading to the initiation of cell death and subsequent release of molecules such as ROS that drive the destruction of the cell [32] . Multiple sources and types of ROS are involved in HR development, and it is generally believed that these are directed against pathogens [33] . Mitochondria are among the multiple organelles that contribute to ROS production. Mutants defective in mitochondrial ROS (mROS) generation exhibit enhanced disease susceptibility to specific fungal and bacterial pathogens [34] . All these studies point to a positive regulatory role of mitochondria during immune responses through ROS generation. Intriguingly, our mutant analysis of Atpam16 alleles suggests that the positive role of mitochondria in ROS production is negatively regulated. Mutations in Atpam16-1 and Atpam16-2 enhance snc1 -mediated autoimmunity ( Figs 1 and 8 ). Single mutants Atpam16-1 , Atpam16-2 and Atpam16l display an enhanced disease resistant phenotype and higher level of PR-1 and PR-2 expression ( Fig. 7b–d ). Atpam16 single mutants also exhibit elevated ROS level ( Fig. 7e,f ). These observations suggest that AtPAM16 functions in negative regulation of plant immunity through repressing mROS production. As AtPAM16 is part of the mitochondrial protein import motor, this regulatory role is probably not direct. We propose that AtPAM16 is involved in the import of a nuclear-encoded negative regulator of plant immunity into the mitochondrial matrix, along with other protein targets. This negative regulator is responsible for repressing processes such as excessive mROS production, which may lead to autoimmunity or unwanted cell death that would be detrimental to the plant ( Fig. 9a ). Mutations in AtPAM16 may therefore attenuate the import of this negative regulator, leading to enhanced immunity ( Figs 7 and 9b ). 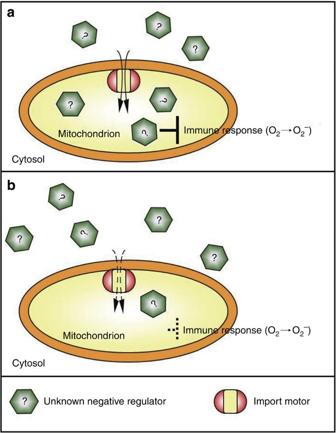Figure 9: Model of AtPAM16 as a subunit of mitochondria inner membrane import motor for negative regulation of plant immunity. (a) AtPAM16 normally facilitates import of an unknown negative regulator (?) into mitochondria during an immune response. This inhibition helps to prevent autoimmunity due to uncontrolled immune response, such as over-production of ROS. (b) With a mutation in AtPAM16, this negative regulator cannot be fully imported into mitochondria, thus leading to autoimmunity and ROS accumulation due to insufficient repression. Partial import of this negative regulator can still be achieved through AtPAM16L. Figure 9: Model of AtPAM16 as a subunit of mitochondria inner membrane import motor for negative regulation of plant immunity. ( a ) AtPAM16 normally facilitates import of an unknown negative regulator (?) into mitochondria during an immune response. This inhibition helps to prevent autoimmunity due to uncontrolled immune response, such as over-production of ROS. ( b ) With a mutation in AtPAM16, this negative regulator cannot be fully imported into mitochondria, thus leading to autoimmunity and ROS accumulation due to insufficient repression. Partial import of this negative regulator can still be achieved through AtPAM16L. Full size image In summary, the plant mitochondria inner membrane import motor AtPAM16 was identified as an important contributor to R protein-mediated immunity, as well as an essential protein in plant survival. This work highlights the significance of negative regulation of mitochondrial activity in plant immunity. Future identification of the AtPAM16 targets will reveal further mechanistic details of how this negative regulation is achieved. Plant growth conditions and mutant screens All plants were grown in climate-controlled chambers under long day conditions (16 h light/8 h dark cycle) at 22 °C. Approximately 10,000 mos4 snc1 mutant seeds were treated with 20 mM ethyl methanesulfonate (EMS) for 18 h. Roughly 50,000 M2 plants representing ~2,500 M1 families were grown on soil and screened for snc1 -like morphology. Seeds of putative mutants were plated on 1/2 MS medium and tested for constitutive pPR2-GUS reporter gene expression by GUS staining. Mutants with constitutive GUS staining were further analysed by H . a. Noco2 infection. Gene expression analysis About 0.07 g tissue was collected from 2-week-old seedlings grown on 1/2 MS medium and RNA was extracted using the Totally RNA kit (Ambion,). Superscript II reverse transcriptase (Invitrogen) was used to reverse transcribe 0.4 μg total RNA to generate cDNA. cDNA samples were initially normalized with ACTIN by real-time PCR using the QuantiFAST SYBR Green PCR kit. The cDNA was subsequently amplified by PCR using 94 °C for 2 min and cycles of 94 °C for 20 s, 58 °C for 30 s and 68 °C for 1 min. The sequences of primers used are: PR-1 F, 5′-GTAGGTGCTCTTGTTCTTCCC-3′ and PR-1 R, 5′-CACATAATTCCCACGAGGATC-3′; PR-2 F, 5′-GCTTCCTTCTTCAACCACACAGC-3′ and PR-2 R 5′-CGTTGATGTACCGGAATCTGAC-3′; Actin-1- F, 5′-CGATGAAGCTCAATCCAAACGA-3′ and Actin-1- R, 5′-CAGAGTCGAGCACAATACCG-3′. Pathogen infections Infection of H.a. Noco2 was performed on 2-week-old soil-grown seedlings sprayed with a concentration of 10 5 spores per ml of water. The inoculated seedlings were subsequently kept in a growth chamber with high humidity (~80%) at 18 °C under 12 h light/12 h dark cycle for 7 days before the growth of H .a. Noco2 was quantified by counting spores. For infections with P.s.m. ES4326, 5-week-old soil-grown plants were infiltrated with bacterial suspension (OD 600 =0.0005) in 10 mM MgCl 2 . Leaf punches were taken at day 0 and day 3. Colony-forming units were determined after serial dilution and bacterial incubation at 28 °C on LB plates [5] . Positional cloning and Illumina whole-genome sequencing Triple mutant muse5-1 mos4 snc1 plants were crossed with WT L. erecta . Crude mapping was performed on F2 plants homozygous for muse5-1 and fine mapping was performed on F3 plants derived from F2 plants heterozygous for muse5-1 and homozygous for mos4 and snc1 . Both the phenotype and genotype of the recombinants were confirmed in the next generation. The markers used to map muse5-1 were designed according to the insertion and deletion polymorphisms between the genomic sequences of Col and Ler ecotypes, provided by Monsanto on TAIR ( http://www.arabidopsis.org ). Once the muse5 mutation was narrowed down to a small region of ~1 Mb, the genomic DNA of seedlings of the muse5-1 mos4 snc1 genotype from the mapping population were sequenced with Illumina whole-genome sequencing following the NEB Instruction Manual of ‘NEB Next DNA Library Prep Master Mix Set for Illumina’. Briefly, the purified genomic DNA was sonicated into fragments of ~300 bp. which were set to end-repair, dA-tailing and adaptor ligation. After removal of unligated adaptors, the ligated DNA was enriched by PCR to create a genomic DNA library. Then, the genomic DNA library was sequenced using an Illumina Genome Analyzer. After comparison with WT genomic sequence, the mutations within the flanking area were selected for further analysis. The sequences of primers for PCR are: P1, 5′-AATGATACGGCGACCACCGAGATCTACACTCTTTCCCTACACGA-3′; P2, 5′-CAAGCAGAAGACGGCATACGAGCTCTTCCGATCT-3′. Transgenic complementation A transgenic complementation experiment was conducted to confirm that the mutation identified in At3g59280/TXR1 is muse5-1 . Full-length At3g59280/TXR1/AtPAM16 genomic DNA including 1,067 bp of native promoter sequence was amplified by PCR, cloned into the pCAMBIA1305 vector and transformed into muse5-1 mos4 snc1 plants by the floral dipping method [35] . Transgenic plants from the T2 generation were selected on 1/2 MS plates containing 50 mg ml −1 of hygromycin to identify homozygous lines. The construct used for TXR1/MUSE5/AtPAM16–GFP analysis was created in the same way but with a vector containing a GFP tag. Seeds of txr1-1 were generously provided by Dr Wolf-Rüdiger Scheible. For allelism test between txr1-1 and muse5-1 , txr1-1 was crossed with muse5-1 mos4 snc1 to generate F1. Morphologic phenotypes of F1 plants were examined. Confocal microscopy Confocal images of AtPAM16 – GFP and mt-CFP transgenic seedlings were obtained with a Leica SP5 confocal microscope (Leica GmbH, Wetzlar, Germany) at 488 nm excitation for GFP (500–540 nm emission, HyD3 detector), at 548 nm excitation for CFP (465–485 nm emission) and at 561 nm excitation for the detection of propidium iodide (600–640 nm emission), which was used at a concentration of 0.05% in H 2 O for staining cell walls. Yeast plasmids Wild-type TXR1/MUSE5 cDNA was PCR-cloned into yeast expression vector p425-GPD, using Bam HI and Sal I restriction sites for inserting AtPAM16 behind the GPD promoter. The previously created pam16-1 mutant was kindly provided by Dr Peter Rehling [12] . Mitochondria isolation and proteinase K digestion assay Mitochondria from AtPAM16–GFP transgenic plants were isolated according to a previously established procedure ( http://www.edvotek.com/Plants ). Briefly, 2-week-old plate-grown seedlings (5 g) were harvested and ground to a fine powder in liquid nitrogen and mixed with 10 ml cold lysis buffer (20 mM Tris-HCI, pH 7.4, 25% glycerol, 20 mM KCI, 2 mM EDTA, 2.5 mM MgCI 2 , 250 mM sucrose and 1 mM PMSF). The homogenate was filtered through a 95-μm and 40-μm nylon mesh sequentially. The flow-through was spun at 4 °C, 700 g for 10 min to pellet the nuclei and cell debris. The supernatant was transferred and centrifuged at 10,000 g for 10 min at 4 °C. The pellet at the bottom is enriched with intact mitochondria. The pellet was further washed using suc washing buffer (0.3 M sucrose, 10 mM Tris, 0.2% BSA) and centrifuged at 10,000 g for 10 min at 4 °C to obtain relatively pure mitochondria. The isolated mitochondria were resuspended in 100 μl of 0.4 M Suc, 50 mM Tris, 3 mM EDTA, 0.1% ( w / v ) BSA, pH 7.5. The mitochondria suspension was further subjected to 10 mg ml −1 proteinase K digestion. Samples were incubated on ice for 10, 20, 30 and 40 min individually before adding 35 μl 4 × Laemmli loading buffer and heated at 95 °C for 5 min. Sonication-disrupted mitochondria solution was used as control for proteinase K digestion. The full western blots are shown in Supplementary Fig. S1 . Cryofixation immune-gold labelling for TEM AtPAM16–GFP transgenic plants were used in cryo-TEM for subcellular localization. Seven-day-old seedlings were high-pressure-frozen in 1-hexadecene in B-type sample holders (Ted Pella) using a Leica HPM-100. Samples were freeze-substituted in 0.1% uranyl acetate, 0.25% glutaraldehyde and 8% dimethoxypropane in acetone for 5 days, then brought to room temperature and infiltrated with LR white resin (London Resin Company) over 4 days. Immunolabeling was performed according to McFarlane et al. [36] , using 1/100 anti-GFP (Invitrogen A6455) and 1/100 goat-anti-rabbit conjugated to 10 nm gold (Ted Pella). Samples were viewed using a Hitachi 7600 TEM at 80 kV accelerating voltage with an AMT Advantage CCD camera (Hamamatsu ORCA). AtPAM16–GFP signal was quantified relative to background by counting the number of gold particles per μm 2 of mitochondria relative to the gold per μm 2 of other cellular contents (cytoplasm, other organelles and cell wall) using ImageJ. Mean gold per μm 2 was compared between mitochondria and the rest of the cell in AtPAM16–GFP and WT without the transgene using ANOVA ( n =81) measurements from eight independent seedlings from two independent transgenic AtPAM16–GFP lines, and 94 measurements from WT. Creating mutants To identify the Atpam16-1 single mutant, Atpam16-1 mos4 snc1 was crossed with WT containing pPR2-GUS . F2 plants were genotyped for the Atpam16-1 , mos4 and snc1 loci by genotype-specific PCR. Lines homozygous for Atpam16-1 without mos4 and snc1 mutations were regarded as Atpam16-1 single mutants. Lines homozygous for Atpam16-1 and snc1 with no mos4 mutation were kept as Atpam16-1 snc1 double mutants. T-DNA insertion mutant Atpam16l was obtained from the Arabidopsis Biological Resource Centre (ABRC). Plants homozygous for the T-DNA insertions were identified by PCR. To create the Atpam16-1 Atpam16l double mutant, Atpam16-1 single mutant was crossed with Atpam16l . In the F2 generation, ~200 plants were genotyped by PCR. The Atpam16-2 snc1 and Atpam16l snc1 double mutants were obtained by crossing Atpam16-2 or Atpam16l to snc1 and the double mutants were identified in F2 by genotyping. DAB staining DAB staining was performed on 2-week-old seedlings grown on 1/2 MS medium, following a previously described procedure. [37] Briefly, the seedlings were soaked with 2 ml DAB solutions (1 mg ml −1 DAB, 0.05% v / v Tween 20 and 10 mM sodium phosphate buffer (pH 7.0)) in a 24-well tissue culture plate and vacuumed for 2 minutes before incubating on an orbital shaker. After 1-hour incubation, the staining solution was removed and the samples were destained with 95% ethanol and examined by microscopy for brown deposition. Oxidative burst detection ROS production from leaves was measured with a previously reported luminol-based assay [38] . In brief, plants were grown in climate-controlled chambers under 12 h light/12 h dark cycles at 22 °C. Leaves of 4-week-old soil-grown plants were sliced into ~1 mm segments and floated in wells overnight on H 2 O under light. H 2 O was replaced with reagent containing luminol, peroxidase and flg22. ROS released by leaf tissue was detected by luminescence of luminol. How to cite this article: Huang, Y. et al. Mitochondrial AtPAM16 is required for plant survival and the negative regulation of plant immunity. Nat. Commun. 4:2558 doi: 10.1038/ncomms3558 (2013).